Neural circuits in the brain that are activated when mitigating criminal sentences In sentencing guilty defendants, jurors and judges weigh 'mitigating circumstances', which create sympathy for a defendant. Here we use functional magnetic resonance imaging to measure neural activity in ordinary citizens who are potential jurors, as they decide on mitigation of punishment for murder. We found that sympathy activated regions associated with mentalising and moral conflict (dorsomedial prefrontal cortex, precuneus and temporo-parietal junction). Sentencing also activated precuneus and anterior cingulate cortex, suggesting that mitigation is based on negative affective responses to murder, sympathy for mitigating circumstances and cognitive control to choose numerical punishments. Individual differences on the inclination to mitigate, the sentence reduction per unit of judged sympathy, correlated with activity in the right middle insula, an area known to represent interoception of visceral states. These results could help the legal system understand how potential jurors actually decide, and contribute to growing knowledge about whether emotion and cognition are integrated sensibly in difficult judgments. Philosophers, psychologists and legal scholars have long debated whether mercy, sympathy and compassion should reduce moral culpability of legal defendants. People do have negative emotional responses to a wide range of situational factors that are not normatively justifiable because they are not considered evidence, or appeal to 'prejudices and sympathy', which jurors are typically instructed to ignore, for example, gruesome crime scene pictures lead to more mock jury convictions when they are in colour (compared with black and white [1] ). Other studies show that evidence that provides negative emotions leads to more punitive judgments [2] . A mock trial study reported that jurors found a defendant less guilty when they heard a defense attorney urging sympathy for the defendant [3] . Studies of moral cognition in hypothetical non-legal scenarios have revealed the increased activity in emotion-related brain regions (that is, insula, amygdala and orbitofrontal cortex) and decreased activity in cognitive processes (that is, dorsolateral prefrontal and parietal areas) when participants contemplated morally charged actions, such as a trolley dilemma involving killing lives of some people to save others [4] . Other studies indicate that people do sometimes punish norm violators in non-legal or legal situations, driven by moral judgments in which negative emotional reactions have a critical role [5] , [6] . Prosocial emotions, such as sympathy, also influence decision making (for example, charitable giving) [3] ; however, there is currently no direct cognitive and neural evidence for how sympathy is translated into legal outcomes. All these studies raise an important question of whether moral judgments and accompanying emotions are used reasonably (as legal rules require) or not. Neuroscience is now entering this debate about defendants, but very little is known about whether mental activity of juries and judges conforms to legal principles. The case we explore here is 'mitigating circumstances', a rare case where emotions, such as sympathy, are allowed to influence juror judgment. The legal domain is unusual because it may be especially challenging to map emotions into numerical legal outcomes. This difficulty is found in studies of hypothetical punitive damages in tort cases, which not only show that jurors typically agree on moral outrageousness of actions, but also show large disagreement about how outrage is mapped to punitive dollar awards [7] , [8] . Weighing mitigation puts an unusual burden on people ( qua jurors) to have appropriate emotional sympathetic reactions, then encode their emotions into prison years. Uncovering the cognitive and neural mechanisms of sympathy that motivate mitigation will inform the role of emotion in jurors' decision process, and perhaps the ultimate policy issue of what role emotional evidence can and should have in trials. Understanding the neuroscientific basis of legal mitigation adds to a basic understanding of moral neuroscience. Neural evidence could also advance theory and practice of law, as so little is known about whether the mental activity of juries and judges conforms to normative legal principles [9] . In summary, our results revealed that sympathy activated brain regions associated with mentalising and moral conflict, including dorsomedial prefrontal cortex (DMPFC), precuneus and temporo-parietal junction (TPJ). Sentence mitigation also recruited these sympathy regions, uncovering neural evidence for a close relationship between sympathy and mitigation. Furthermore, individual differences on the inclination to mitigate were reflected in differential middle insula activity. These findings do not just contribute to the field of neuroscience, but could help lawmakers to understand jurors' decision making and their individual differences in trials. Sympathy and no-sympathy scenarios. We measured brain activity using functional magnetic resonance imaging (fMRI) while subjects are making hypothetical sentence reduction decisions, in dramatic scenarios adapted from actual murder cases. Sympathy-related brain activity was collected during reading circumstances pertaining to defendants' crimes ( Fig. 1a ). Only actual Japanese murders were used, so the crime was serious, uniform across trials and lifelike. This simple design was chosen to generate engagement and limit nuisance brain activity due to subtle differences in crimes and plausibility of artificially created scenarios. 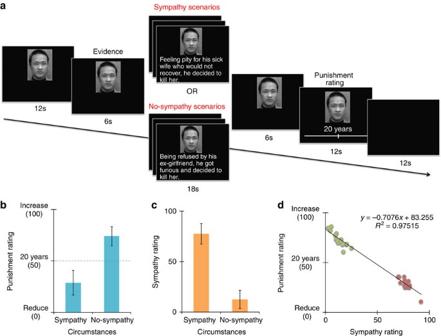Figure 1: Task design and behavioural performance. (a) Study paradigm. (b) Mean punishment ratings for sympathy and no-sympathy trials (n= 22, pairedt-test,t21=−18.94,P<0.001). (c) Mean sympathy ratings for sympathy and no-sympathy trials (n= 22, pairedt-test,t21=11.82,P<0.001). (d) Correlation between sympathy and punishment ratings for sympathy stories (red circles) and no-sympathy stories (green circles). Error bars indicate s.d. Figure 1: Task design and behavioural performance. ( a ) Study paradigm. ( b ) Mean punishment ratings for sympathy and no-sympathy trials ( n = 22, paired t -test, t 21 =−18.94, P <0.001). ( c ) Mean sympathy ratings for sympathy and no-sympathy trials ( n = 22, paired t -test, t 21 =11.82, P <0.001). ( d ) Correlation between sympathy and punishment ratings for sympathy stories (red circles) and no-sympathy stories (green circles). Error bars indicate s.d. Full size image Mitigating circumstances were of two types: those that would induce sympathy and those that would not. The sympathy scenarios included desperate situations of defendants suffering from domestic violence, disease or poverty. Figure 1a gives one example of each type. The intentionality and severity of the murders were matched between conditions (see Supplementary Methods ). After reading about the circumstances, subjects decided how much they would change the sentence given for the defendant (initially 20 years) if they were on a jury. After scanning, subjects were again presented with the same scenarios and asked to rate how much sympathy they felt for the defendant, using a visual analogue scale. Sympathy and punishment ratings. The sympathy manipulation is internally valid because participants gave significantly higher sympathy ratings to those defendants with sympathy circumstances compared with those with no-sympathy circumstances ( n = 22, paired t -test, t 21 =−18.94, P <0.001, Fig. 1b ). They also reduced sentences much more in sympathy circumstances ( n = 22, paired t -test, t 21 =11.82, P <0.001, Fig. 1c ). Unsurprisingly, sympathy and punishment (sentence length) were highly negatively correlated ( n = 32 stories, linear regression analysis, P < 0.001, R 2 =0.97, Fig. 1d ). fMRI results were analysed using standard generalized linear model regression techniques (see Methods ). A short block design was used where regressors were included for the various events of the trials ( Fig. 1a ). Interaction terms corresponding to punishment and sympathy ratings interacted with trial onsets that were added as parametric regressors. Brain regions associated with sympathy scenarios We first analysed brain areas exhibiting a stronger response in sympathy scenarios than no-sympathy scenarios. Precuneus, left TPJ and DMPFC showed larger activities for sympathy than for no-sympathy scenarios ( n = 22, one-sample t -test, Table 1 ). These regions are related to mentalization and sympathy as discussed below in detail, which confirms that the experimental manipulation of sympathy produced results consistent with the sympathy ratings data. Table 1 Areas exhibiting a stronger response in sympathy scenarios. Full size table Brain regions associated with punishment and sympathy We then searched for brain regions that responded, during the description, to the subjects' trial-by-trial ratings of sympathy and their amounts of punishment reduction. Activity in precuneus, DMPFC and left TPJ were correlated with sympathy ( P <0.05, small-volume-corrected, Fig. 2 , Supplementary Table S1 ). Signal increase in precuneus and DMPFC were also associated with the reduction of punishment ( P <0.05, small-volume-corrected, Fig. 2 : note that a small TPJ region was also activated in sentence reduction, but only with k =6 voxels). Thus, precuneus and DMPFC were commonly activated by both sympathy and reduction of punishment. Sentence reduction was also associated with activity in anterior cingulate cortex (ACC). All regions showing a whole-brain correlation at P <0.001 are listed in Supplementary Tables S1 and S2 . 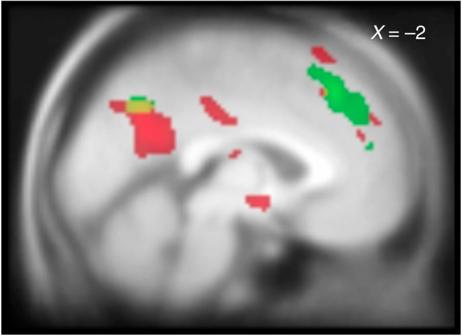Figure 2: Brain regions activated during trial-by-trial sympathy and punishment reduction. Regions in which activity correlated with parametric regressors of increasing sympathy (green) and reduced punishment (red). Common areas were found in precuneus (yellow). The image is shown atP<0.001 (uncorrected;n= 22, one-samplet-tests). Figure 2: Brain regions activated during trial-by-trial sympathy and punishment reduction. Regions in which activity correlated with parametric regressors of increasing sympathy (green) and reduced punishment (red). Common areas were found in precuneus (yellow). The image is shown at P <0.001 (uncorrected; n = 22, one-sample t -tests). Full size image Brain regions associated with an inclination to mitigate Next, we constructed an individual-specific measure of an inclination to mitigate, by reducing sentences, as a function of sympathy. This measure comes from a simple linear regression on each individual's decisions: punishment= b 0 + b 1 *sympathy+error [10] . A measure of an inclination to mitigate, the reduction in sentence per unit of sympathy, was given by the b 1 coefficient of the regression. This number represents a complex mapping from an emotional response to a number representing prison time for a defendant (a years-per-emotion coefficient). These b 1 coefficients were negative for all subjects (mean=−6.5±0.2, linear regression analysis, all P <0.001), indicating that the feeling of sympathy did correlate with reduction of punishment, but to different degrees across subjects. A negative linear regression between the individual-specific b 1 coefficient and blood oxygenation level-dependent responses in sympathy minus no-sympathy trials found activity in the right middle insula ( P <0.05, small-volume-corrected, Fig. 3 ). Individuals who had larger activities in the insula when reading circumstances showed higher tendencies to mitigate, reducing sentencing years more as their sympathy increased. 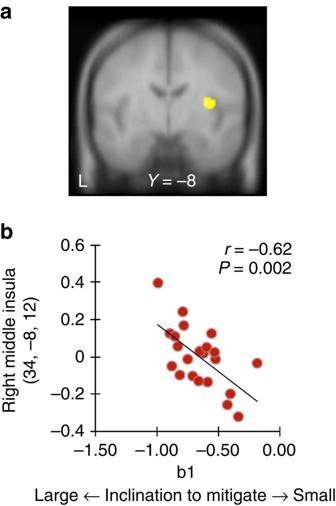Figure 3: Individual differences in inclination towards mitigation. Activation in right middle insula in the contrast sympathy minus no-sympathy trials (a, MNI 34/−8/12;n= 22, one-samplet-test,P=0.023, small-volume-corrected) correlated with participant-wise coefficient of mitigation (b,n= 22, Pearsonr=−0.62,P=0.002). Figure 3: Individual differences in inclination towards mitigation. Activation in right middle insula in the contrast sympathy minus no-sympathy trials ( a , MNI 34/−8/12; n = 22, one-sample t -test, P =0.023, small-volume-corrected) correlated with participant-wise coefficient of mitigation ( b , n = 22, Pearson r =−0.62, P =0.002). Full size image Comparison of activity during judgments of sympathy, and sentence reduction, suggest that activity in DMPFC (also known as paracingulate), precuneus (also known as posterior cingulate) and TPJ reflect a judgment-action circuit, which is illustrated in Fig. 2 . Strength of sympathy judgments is associated with activity in DMPFC, precuneus and TPJ. DMPFC is involved in general mentalising [11] and is active when empathizing [12] or sympathizing [13] with others in pain. Precuneus has been linked to subjective perspective taking [14] , [15] , [16] . TPJ is also commonly identified as a part of a theory-of-mind circuit [17] , including mentalising about intentions [18] , and was activated in one study on judging innocence of intentions of people who caused harm [19] . This suggests that the sympathy judgment is an engagement with a reasoned simulation of what the defendant was thinking when committing the crime or how most people would judge the normative basis for mitigation. Note that although precuneus and TPJ can each be activated by non-social demands as well (for example, attention reorienting [20] ), they are rarely co-activated as a group unless social cognitive demands are present. Regions activated by the punishment reduction judgment include a large region of precuneus and smaller regions in DMPFC and ACC. As noted, precuneus has been linked to simulation on the self to understand others, and is also active when compassionating [21] and forgiving others [22] . The activation in this area is correlated with more iterated steps [23] and higher-value [24] strategic thinking in game theory tasks. Note that both feelings of sympathy and judged mitigation of punishment were encoded in activity in precuneus. This overlapping activity suggests that the precuneus may be a region that accepts emotional judgment input and maps it into concrete punishment actions. ACC is a region now thought to be activated by negative affect [25] , [26] , positive reward [27] and cognitive control [26] , [28] . In our context, mapping emotional sympathy into numerical sentencing requires high-level executive function by weighing negative affective reaction to murder, positive sympathy for the murder's mitigating circumstances and exerting cognitive control to choose numerical punishments that weigh these emotions consistently. Smaller regions in caudate also showed differential activation in response to punishment reduction ( Supplementary Table S2 ). Caudate activity is consistent with the hypothesis that sentence reduction is encoded as a special kind of prosocial 'charity' (as mitigation is like giving to charity [29] ), as other prosocial choices activate the caudate too [30] . One fMRI study elicited punishment judgments in artificial scenarios varying offender culpability [6] and reports right DLPFC activity associated with responsibility judgments. We speculate that the absence of right DLPFC activation in our study is because there is no doubt about the defendants' guilt, so the most morally burdensome question of guilt versus innocence is resolved (right DLPFC is discharged from jury duty, so to speak). Activity then shifts to areas generally associated with moral and cognitive conflicts instead (DMPFC, precuneus and ACC). The individual difference analysis showed that activity in the right mid-insula was related to the individual differences on the inclination to mitigate (mapping sympathy to sentences). Middle/posterior insula has been suggested to encode economic inequity [31] , norm violation [32] , somatosensory representation [33] , monitoring internal states [34] and heart rate during a compassionate state [35] . These types of interoceptive processing in middle insula suggest that it is sensitive to emotions linked to sociality. Our study provides unusual evidence of this processing associated with a unique high-impact social judgment that affects others. The identified brain activity provides new insight into the capacity of the average brain to translate sympathetic feelings into appropriate legal action. A plausible neuro-legal standard is that the influence of sympathetic reaction on difficult sentencing should recruit brain areas that process sympathy judgments in general, as well as areas that encode difficult decision conflict. Activity in these 'sympathy' regions is evident in our study when judging sympathy alone, and in choosing sentence mitigation. However, not every brain maps sympathy to prison sentences in the same numerical way (as reflected in differential mid-insula activity). Differences in these brain circuits between individuals, suggest that differential juror responses might need to be considered unequally. There is also mixed evidence about the normative basis of legal judgment, including a recent finding that judges' decisions are affected by timing of meals [36] . The current finding would also contribute to the attribution literature on situational correction, as there has not been any fMRI work on this. People often attribute behaviour to the corresponding personal disposition, which is, yet, corrected based on situational inducements too [37] . This is an apt psychological function behind mitigating circumstances that is to make someone less culpable, and the revealed brain activity might be associated with this type of situational correction. Finally, we note that many legal principles treat emotional responses as likely to be prejudicial and prone to inflammatory manipulation (that is, an ideal juror would suppress them and legal rules limit their influence). Weighing mitigating circumstances during sentencing ( after a verdict) represents an unusual case in which emotional sympathy judgment is actually required. Japanese criminal law, for example, requires that the decision among these sentences be based on mitigating circumstances [38] . Ironically, the fact that sympathy is clearly evident in brain activity, and influences sentence mitigation (as it should), raises interest in the opposite question: can people also suspend emotions when the law instructs them to? More generally, a deeper understanding of the brain could help figure out how highly evolved brain structures, which were sculpted to maintain order in small-scale ancestral societies, can be put to work under modern legal rules in much more challenging cases to create modern justice. Participants A total of 26 right-handed healthy subjects (12 males; mean age=21.5±1.8 (s.d.) years) participated in the study. All subjects had normal or corrected-to-normal vision, no history of neurological or psychiatric disorder and were not taking medications that interfere with the performance of fMRI. The study was approved by the Ethics and Radiation Safety Committee of the National Institute of Radiological Sciences (Chiba, Japan). Data from four participants were discarded owing to excessive movement (three subjects) and sleep (one subject). The data from 22 subjects (11 males; mean age=21.5±1.9 (s.d.) years) were included and analysed. Stimuli and the task A total of 32 faces of defendants and criminal acts were prepared in the study. Faces were drawn from a set of Asian face stimuli developed by CAS-PEAL face database [39] . Pilot participants ( n =30) rated attractiveness for each faces using an 11-point scale of −5 (not attractive at all) to +5 (very attractive). The average attractiveness for 32 faces was 0.15±0.70. All criminal acts were the pure murder cases, which were modified from real stories taken from a precedent search engine provided by Supreme Court of Japan ( www.courts.go.jp ) and from news articles on the web. We prepared 32 scenarios and consulted a judicial expert for advice on how externally valid the scenarios were. Each scenario composed of the fact (when, where and to whom) and the circumstance (why the defendant committed the murder). Half of the scenarios would induce sympathy for the defendants who suffer from domestic violence, death to disease or poverty (sympathy scenarios), and the other half that would not (no-sympathy scenarios). Responsibility, intentionality and severity of crime were matched between scenarios (see Supplementary Methods for all scenarios used in the study). Subjects were instructed to judge crimes as if they were jurors (lay judges). Before entering the scanner, subjects read each criminal case and were asked to indicate if they have known them through media. The aim of this session was to ensure and ease comprehension in the scanner that constrain duration of presenting each scenario. During the fMRI task, subjects read each scenario and rated how much they would like to reduce or increment the sentence (all 20 years) given for the defendant using a VAS (with scores ranging from 0=reduce as much as possible to 100=increment as much as possible, and 50=given sentence of 20 years; Fig. 1a ). We chose a sentence of 20 years as a reference point, based on a sentencing guideline in Japan that gives 20 years in prison to a person who commits murder. Defendants' faces were presented together with the scenarios in order to make the experimental setting more realistic and to help participants to dedicate to the study. They completed two sessions, and each session contained 8 sympathy and 8 no-sympathy scenarios, 16 trials in total. The presentation of each scenario within a session was pseudorandomized. The order of sessions and the combination of faces and circumstance types were counterbalanced between subjects. After the scan, subjects were shown the same scenarios again to rate how much they felt sympathy for the defendants using a VAS (with scores ranging from 0=having no sympathy to 100=having sympathy very much). They were also asked to fill out Interpersonal Reactivity Index (IRI), a self-report measure of dispositional empathy. fMRI data acquisition The functional imaging was conducted using a GE 3.0 Tesla Excite system to acquire gradient echo T2*-weighted echoplanar images with blood oxygenation level-dependent contrast. Each volume comprised 35 transaxial contiguous slices with a slice thickness of 3.8 mm to cover almost the whole brain (flip angle, 75; echo time, 25 ms; repetition time, 2000 ms; matrix, 64*64; and field of view, 24×24 cm 2 ). fMRI data preprocessing Image analysis was performed using SPM8 (Wellcome Department of Imaging Neuroscience, Institute of Neurology, London, UK), except for the overlay image shown in Fig. 2 that was created using the MRIcron software ( http://www.sph.sc.edu/comd/rorden/mricron/ ). All volumes were realigned to the first volume of each session to correct for subject motion and were spatially normalised to the standard space defined by the Montreal Neurological Institute (MNI) template. After normalisation, images were spatially smoothed using a Gaussian kernel with a full-width-at-half-maximum of 8 mm. Intensity normalisation and high-pass temporal filtering (using a filter width of 128 s) were also applied to the data. Generalized linear model For the primary whole-brain analyses, two modelling approaches were used. In the first approach, trials from each of the sympathy and no-sympathy circumstances were modelled as separate conditions. This allowed separate estimation of the evoked response for each of the conditions at each voxel. The model also included regressors for face, criminal evidence, punishment, and fixation, as well as six head-motion parameters as regressors of no interest. We first calculated a first-level single-subject contrast for reading sympathy minus no-sympathy circumstances. Then, we calculated a second-level group contrasts using a one-sample t -test. In the second approach, all trials from reading circumstances modelled using a single condition (that is, overall task-related activation), and two additional orthogonal parametric regressors were included representing (a) the amount of reducing punishment and (b) the level of sympathy rating. We first calculated first-level single-subject contrasts for reading circumstances modulated by reducing punishment and for reading circumstances modulated by sympathy rating. Then, we calculated second-level group contrasts using one-sample t tests on the single-subject contrasts to identify brain regions whose activation correlated with the amount of reducing punishment and the sympathy rating. A statistical threshold of P <0.05 corrected for multiple spatial comparisons across the whole brain at cluster level was used, except for a priori hypothesized regions that were voxel thresholded at P <0.001 uncorrected (only clusters involving k >10 or more contiguous voxels were reported [40] ). Small volume correction (a 10-mm radius sphere) was used on a priori regions of interest: DMPFC/ACC, precuneus/posterior cingulate cortex, TPJ and the insula. How to cite this article: Yamada, M. et al . Neural circuits in the brain that are activated when mitigating criminal sentences. Nat. Commun. 3:759 doi: 10.1038/ncomms1757 (2012).